N-Heterocyclic carbene-catalyzed enantioselective synthesis of planar-chiral cyclophanes via dynamic kinetic resolution 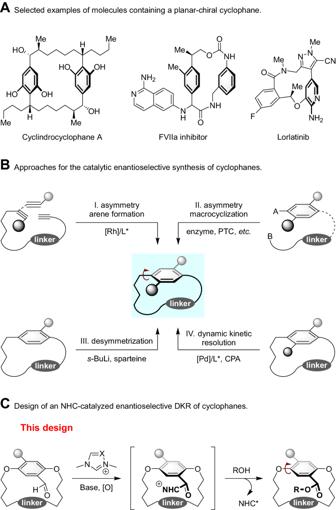Fig. 1: Importance of cyclophanes and the enantioselective synthesis. ASelected examples of molecules containing a planar-chiral cyclophane.BApproaches for the catalytic enantioselective synthesis of cyclophanes.CDesign of an NHC-catalyzed enantioselective DKR of cyclophanes. Planar-chiral cyclophanes have gained considerable concerns for drug discovery due to their unique conformational strain and 3D structure. However, the enantioselective synthesis of planar-chiral cyclophanes is a long-standing challenge for the synthetic community. We herein describe an N-heterocyclic carbene (NHC)-catalyzed asymmetric construction of planar-chiral cyclophanes. This transformation occurs through a dynamic kinetic resolution (DKR) process to convert racemic substrates into planar-chiral macrocycle scaffolds in good to high yields with high to excellent enantioselectivities. The ansa chain length and aromatic ring substituent size is crucial to achieve the DKR approach. Controlled experiments and DFT calculations were performed to clarify the DKR process. Macrocycles exhibit unique properties including shape diversity, conformational pre-organization, and conformational flexibility, compared to small-sized rings, particularly, five- to seven-membered rings [1] , [2] . The large surface area and tunable conformation of macrocycles increase the likelihood that the macrocycle will make meaningful contact with a biological target [1] , [3] . The compilation of macrocyclic small molecule screening libraries is critical to success when challenging, underexploited, or poorly “druggable” biological targets, such as lorlatinib, are involved [1] , [4] . Cyclophanes, which are molecules with an aromatic scaffold bearing a cross-linked chain, also called an ansa chain, are a subset of macrocycles [5] , [6] , [7] . Notably, cyclophane with a short ansa chain and bulky aromatic substituents exhibit planar chirality, which arises from the restricted bond flip of the aromatic ring [8] , [9] , [10] . Although planar-chiral cyclophanes are part of small molecule screening collections, these compounds have been increasingly used in drug development [11] , [12] , asymmetric synthesis [13] , and functional materials [14] (Fig. 1A ), and additional planar-chiral cyclophanes could benefit these collections. However, the enantioselective synthesis of planar-chiral cyclophanes represents a formidable challenge to the synthetic community and hampers their widespread inclusion in drug development efforts [15] , [16] . Fig. 1: Importance of cyclophanes and the enantioselective synthesis. A Selected examples of molecules containing a planar-chiral cyclophane. B Approaches for the catalytic enantioselective synthesis of cyclophanes. C Design of an NHC-catalyzed enantioselective DKR of cyclophanes. Full size image Historically, the asymmetric synthesis of cyclophanes relied on chiral pools and chiral auxiliaries [17] , [18] , [19] , [20] , [21] . Asymmetric catalysis now provides access to the enantiopure planar-chiral cyclophanes [16] , as seen in Tanaka’s seminal asymmetric arene formation strategy to produce chiral metacyclophanes via rhodium-catalyzed alkyne cyclotrimerization [22] . Inspired by Tanaka’s pioneering work, several elegant enantioselective inter- and intramolecular [2 + 2 + 2] cycloaddition processes were reported for planar-chiral cyclophane assembly (Fig. 1B , I) [23] , [24] , [25] . In addition, asymmetric macrocyclization strategies have also provided access to planar-chiral cyclophanes [26] , [27] , [28] , [29] , [30] , [31] , [32] . Very recently, Collins [28] , Yang [29] , and Li [30] independently developed enzyme-, chiral phosphoric acid (CPA)- or Pd-catalyzed asymmetric macrocyclization to achieve planar-chiral macrocycles (Fig. 1B , II). In addition to these processes, the desymmetrization is also an attractive method to afford planar-chiral structures. Shibata achieved the enantioselective synthesis of planar-chiral cyclophanes by ortho -lithiation of the achiral cyclophanes (Fig. 1B , III) [33] . The fourth is dynamic kinetic resolution (DKR) of achiral cyclophanes (Fig. 1B , IV). The challenges in generating planar-chiral cyclophanes by a DKR process involve identifying appropriately sized aromatic ring substituents and ansa chain lengths, which will allow rapid racemization of the substrate but limit the bond flip of the aromatic ring in the product. Both components are necessary to ensure the configurational stability of the resulting planar-chiral cyclophanes. In this scenario, Shibata was able to produce the chiral cyclophanes by a double asymmetric Sonogashira coupling of achiral [n, n]paracyclophanes [34] . More recently, Yang demonstrated an elegant CPA-catalyzed asymmetric electrophilic aromatic amination protocol to deliver planar-chiral macrocycles [35] . Despite the previously mentioned straightforward approaches to afford planar-chiral cyclophanes, limitations include variable enantiomeric excess for different substrates, low reaction efficiencies, limited scope, and the use of stoichiometric amounts of chiral reagents. Further, the current protocols are restricted to a handful of catalytic models, and organocatalytic enantioselective synthetic routes are still in their infancy [16] . Consequently, these challenges prompted us to develop a DKR approach to achieve optically pure planar-chiral cyclophanes. Chiral N-heterocyclic carbenes (NHCs) have been widely used as powerful organo-catalysts to access molecular architectures [36] , [37] , [38] , [39] , [40] , [41] , [42] , [43] , [44] . However, most previous reports focused on the synthesis of central chirality, and more recently, axial chirality [45] , [46] , [47] , [48] , [49] . Only recently has successful control of planar-chiral ferrocenes through NHC catalysis been reported by Chi [50] . Herein, we disclose an NHC-catalyzed DKR of racemic cyclophanes by an oxidative esterification reaction to afford the planar-chiral cyclophanes in good to high yields with high to excellent enantioselectivities (Fig. 1C ). We have also demonstrated that our enantioenriched products can be easily converted into diverse planar-chiral scaffolds for potential library inclusion and asymmetric catalysis through cross-coupling reactions. Controlled experiments and DFT calculations were performed to clarify the DKR process. Reaction optimization We set out to explore the DKR of cyclophanes by examining the reaction of [14]paracyclophane 1a with (3,5- di-tert -butylphenyl)methanol 2a in the presence of triazolium NHC as catalyst (Fig. 2 ). The atropisomerism of 1a was observed by variable temperature 1 H NMR experiments (below −50 °C), suggesting a low rotational energy barrier for [14]cyclophane 1a at room temperature. Using 1,8-diazabicyclo[5.4.0]undec-7-ene (DBU) as base, 3,3’,5,5’-tetratert-butyldiphenoquinone (DQ) as oxidant, and THF as solvent, various chiral triazoline NHC catalysts I – VII were initially screened (entries 1–7). The pyrrolotriazolium-derived NHC catalyst I exhibited high conversion but low enantioselectivity, while amino alcohol-derived chiral NHC VII afforded the desired product in good yield with moderate enantioselectivity (entries 1 and 7). The N-substituents of the indanol-derived catalysts have an obvious impact on the enantioselectivity of the reaction, as N-2,4,6-(Me) 3 C 6 H 2 (Mes), N-2,4,6-(Br) 3 C 6 H 2 , or N-C 6 F 5 substituents gave the product in high yield but with poor enantioselectivity (entries 2, 3, and 6). Pleasingly, the enantioselectivity was dramatically increased when bulky N-2,4,6-( i Pr) 3 C 6 H 2 or N-2,4,6-Cy 3 C 6 H 2 [51] substituted indanol-derived NHC IV or V catalyst was used (entry 4–5, 93:7 er). Further base optimization indicated that strong bases, such as DBU and Cs 2 CO 3 , resulted in higher yields compared to relatively weak bases (entries 8–10). Subsequent solvent experimentation demonstrated that THF achieved the highest yields (entries 11–13). Decreasing the catalyst loading was not detrimental to reaction outcomes (entry 14). Interestingly, increase of temperature yielded the product in a higher er (entry 15). The improved enantioselectivity might arise from a faster racemization rate of the substrate, which facilitate the DKR process. The absolute configuration of 3aa was unambiguously determined by X-ray diffraction analysis of its derivative ( vide infra ). Fig. 2: Optimization of the reaction conditions. a Reaction conditions: A mixture of 1a (0.10 mmol), 2a (0.12 mmol), DQ (0.10 mmol), Base (10 mol%), and NHC catalyst (10 mol%) in solvent (2.0 mL) was stirred at room temperature for 24 h, the number in the black circle is the ansa chain length. b Isolated yield. c Determined by HPLC using a chiral stationary phase. d NHC catalyst (5 mol%); the reaction was stirred for 48 h. e The reaction was performed at 40 °C. Full size image Substrate scope With the optimized conditions in hand, we then evaluated the effect of the alcohol, starting with substituents on the phenyl ring of the benzyl alcohol. Regardless of the steric and electronics of the aromatic ring substituents, the desired planar-chiral cyclophanes ( 3ab – 3ad ) were afforded good yield with moderate to good enantioselectivities (Fig. 3 ). When substrates bearing bulkier groups were used, good yields and high enantioselectivities were achieved ( 3ae , 78% yield and 95:5 er). When other cyclic secondary alcohols were evaluated, the corresponding products 3af – 3aj were obtained in 48–78% yield with er ranging from 93:7 – >99:1. Moreover, the benzyl alcohol with a 4-prenyl group was not an appropriate substrate for this reaction under the optimized conditions ( 3ak ). Fig. 3: Evaluation of the effect of various alcohol substrates. a The reaction was performed at room temperature, IV was used as catalyst. b The reaction was performed at 40 °C, V was used as catalyst. Full size image The investigation of ansa chain length and substituent size was conducted using 2e as model substrate (Fig. 4 ). Reducing to 11- or 12-membered ansa chains, the reaction went through a kinetic resolution process, in which planar-chiral products 3be and 3ce were obtained in 86:14 er and 91.5:8.5 er, respectively, while 1c was recovered with 51% yield and 82:18 er. Using a 13-membered ansa chain was feasible, delivering the planar-chiral [13]paracyclophane 3de with moderate yield and good enantioselectivity. Increasing the ansa chain length and using a 15-membered compound was tolerated and gave the product 3ee in 72% yield with a 95:5 er value, while [16]paracyclophane 3fe led to the loss of planar chirality due to the relative low rotation barrier. Fig. 4: Evaluation of the ansa chain length and aromatic ring substituent size. a The reaction was performed at room temperature, IV was used as catalyst. b The reaction was performed at 40 °C, V was used as catalyst. c 0.2 mmol of 2a was used. d The reaction was performed at 50 °C, V was used as catalyst. e The reaction was stirred at room temperature for 24 h, 1k was recovered in 55:45 er, and 1 l was recovered in 50:50 er. Full size image In addition, an examination of the aromatic ring substituent size was performed (Fig. 4 ). 4-H substituted [14]paracyclophane resulted in the loss of planar chirality ( 3ge ), but [14]paracyclophanes bearing chloro, methyl, or iodo groups on the benzene ring allowed the NHC-catalyzed DKR to occur, generating the planar-chiral cyclophanes in good yields and enantioselectivities ( 3he – 3je ). Installment of phenyl or ethynyl groups on the aromatic ring was also tolerated. The products 3ke and 3le were obtained in high er value, and corresponding substrates 2k and 2 l were recovered in low er value, which suggested racemization of the substrates occurred. These results indicate that the DKR of planar-chiral [n]paracyclophanes is highly dependent on ansa chain length and the size of substituents in the aromatic ring, which allows substrate racemization but limits bond flip in the product’s aromatic ring. Encouraged by these results, we continued to explore the scope of [n]paracyclophanes in this NHC-catalyzed DKR reaction. A diverse array of achiral paracyclophanes with a variety of ansa chain lengths and substituents were tested (Fig. 5 ). [13]paracyclophane with a chloro group at the 4-position of the phenyl ring performed well to deliver the corresponding planar chiral product ( 5ae ) in good yield and enantioselectivity. [14] and [15]paracyclophanes bearing different substitutes (vinyl, iodo, ethynyl, phenyl) at the phenyl ring were also accommodated and provided the enantioenriched products ( 5be – 5fe ). Heteroaromatic rings like 3-thienyl could be introduced at the 4-position of the substrates ( 5ge, 5he ). [16] and [17]paracyclophane with 2-naphthyl, benzofuran-6-yl or benzo[b]thiophen-3-yl yielded the produts in high enantioselectivity ( 5ie – 5ke ), as could [18]paracyclophane with benzofuran-6-yl albeit with lower enantioselectivity ( 5le ). In addition, modifications of the ansa chain were also investigated. The yield of [14] and [15]paracyclophane with an ester group or nitrogen-linked ansa chain decreased to 26% and 16% ( 5me, 5ne ), respectively. The decreased yield of 5me probably originated from substrate decomposition under the reaction conditions. [15]paracyclophane with an oxygen-linked ansa chain afforded the product in good yield with high enantioselectivity ( 5oe ). To assess the configurational stability of the planar-chiral products, 3ae in toluene was heated to 110 °C. Notably, HPLC analysis indicated that no racemization of 3ae was observed, even after 7 days at this temperature (see Supplementary Information). Fig. 5: The scope of [n]paracyclophanes. a The reaction was performed at 40 °C. b The reaction was performed at 50 °C. c The reaction was performed at room temperature, 5ge was obtained in 86:14 er. d The reaction was performed at 40 °C, 5ge was obtained in 92:8 er. e The reaction was performed at 40 °C, IV was used as catalyst. Full size image To expand the potential utility of this process, we further manipulated the planar-chiral cyclophane (Fig. 6A ). The ester in 3ae could be reduced with LiAlH 4 to generate benzylic alcohol 6 in 98% yield with only a slight erosion of enantioselectivity. In addition, a Ni-catalyzed cross–coupling reaction of 3ae with diphenylphosphine afforded planar-chiral phosphine 7 in 61% yield with a slight loss of stereochemical integrity due to the vigorous reaction conditions. Moreover, the enantiomerically enriched triazole 8 was obtained by a Sonogashira cross–coupling, desilication, and CuTC-catalyzed click reaction sequence. Finally, 3ae was easily transferred to corresponding pyrene-bearing product 9 in 68% yield and 93:7 er through a Suzuki–Miyara cross–coupling reaction with pyren-1-ylboronic acid. The absolute configuration of 10 was unambiguously determined by X-ray diffraction analysis ( https://www.ccdc.cam.ac.uk/data_request/cif ) (Fig. 6B ). Fig. 6: Derivatizations of the chiral product. A Synthetic transformation of enantioenriched [14]paracyclophane 3ae . Reaction conditions: (i) LiAlH 4 , 0 °C, THF, 2 h. (ii) Ni(dppe)Cl 2 , Ph 2 PH, Et 3 N, DMF, 120 °C, 12 h. (iii) Pd(PPh 3 ) 2 Cl 2 , CuI, TMS-acetylene, Et 3 N, 50 °C, 10 h, THF, 91% yield, 93:7 er. (iv) TBAF•3H 2 O, THF, rt, 4 h, 87% yield, 93:7 er. (v) CuTC, ( R )-Camphor-10-sulfonyl azide, toluene, rt, 4 h, 96% yield, 13:1 dr. (vi) Pd(PPh 3 ) 4 , Na 2 CO 3 , pyren-1-ylboronic acid, 1,4-dioxane, 100 °C, 24 h, 68% yield, 93:7 er. B X-ray of planar-chiral cyclophane 10 . Full size image A postulated mechanism is illustrated in Fig. 7 . The reaction starts from the addition of NHC catalyst IV to aldehyde 1a to generate Breslow intermediate Int-I . Then, the oxidation of Int-I forms acylazolium intermediate Int-II . Finally, the esterification of Int-II with benzylic alcohol 2e delivers the planar-chiral product 3ae and releases the free NHC catalyst IV . Fig. 7 Postulated mechanism of the reaction. Full size image The DKR process originates from the rapid bond flip of the aromatic ring in the two enantiomers ([ S p ]− 1a and [ R p ]− 1a ) and the reaction-rate difference with the addition of NHC catalyst (Fig. 8 , eq 1). To clarify the DKR process, several controlled experiments were conducted. The reaction of [15]paracyclophane 4 f with 2e was performed under standard conditions for 12 h; 5fe was obtained in 48% yield with 90:10 er, and 4 f was recovered as racemates in 40% yield. The result indicates that the racemization of 4k is rapid and not the rate-determined step (Fig. 8 , eq 2). In addition, as illustrated in the investigation of substrate scope, [12]paracyclophane underwent kinetic resolution, thus, enantioenriched 4-phenyl-substituted [12]paracyclophane ( R p )− 11 was treated under the optimized reaction conditions, the reaction proceeds smoothly to deliver ( R p )− 12 in 82% yield with >99:1 er value (Fig. 8 , eq 3). Alternatively, only a trace amount of ( R p )− 12 was obtained by using ent -IV as NHC catalyst (<5% yield), and the ( R p )− 11 was recovered in 89% yield with 97:3 er value (Fig. 8 , eq 4). Further, the reaction of 1a and 2e with ent -IV as catalyst gave a reverse selectivity, suggesting that the ( R p )− 11 was unmatched with ent -IV (Fig. 8 , eq 5). These results indicate that the reaction of NHC catalyst IV to ( R p )- 11 is kinetically favored. Fig. 8 Controlled experiments of the dynamic kinetic resolution process. Full size image To further explore the energy-difference for the addition of NHC catalyst IV to the enantiomers ( S p )- 1a and ( R p )- 1a , a density functional theory (DFT) study was performed using Gaussian 09. 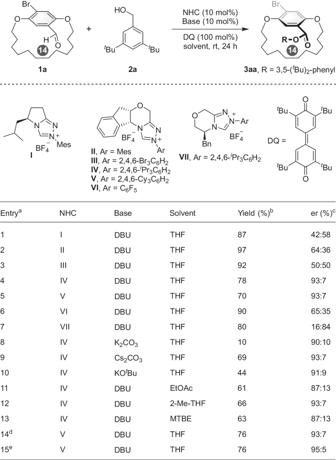Fig. 2: Optimization of the reaction conditions. aReaction conditions: A mixture of1a(0.10 mmol),2a(0.12 mmol), DQ (0.10 mmol), Base (10 mol%), and NHC catalyst (10 mol%) in solvent (2.0 mL) was stirred at room temperature for 24 h, the number in the black circle is theansachain length.bIsolated yield.cDetermined by HPLC using a chiral stationary phase.dNHC catalyst (5 mol%); the reaction was stirred for 48 h.eThe reaction was performed at 40 °C. As illustrated in Fig. 9 , the energy barrier of the addition of NHC catalyst IV to ( R p )- 1a is 3.6 kcal/mol lower than that of ( S p )- 1a ; thus, the addition of NHC catalyst IV to ( R p )- 1a is kinetically favored. Further analysis of transition states TS-( S p )-1a and TS-( R p )-1a using atoms-in-molecules [52] , [53] and noncovalent interactions analyses [54] reveal that the weak interactions in TS-( R p )-1a are stronger than those observed in TS-( S p )-1a , which leads to TS-( R p )-1a having a lower energy barrier. Interactions in TS-( R p )-1a include: seven C–H…π interactions, four C–H…O hydrogen bond interactions, two C–H…N hydrogen bond interactions, one Lp…π interaction, one C–H…Br halogen bond interaction, and ten C–H…H–C van der Waals interactions. Interactions in TS-( S p )-1a include: four C–H…π interactions, three C–H…O hydrogen bond interactions, one C–H…N hydrogen bond interaction, two C–H…Br halogen bond interactions, and nine C-H…H–C van der Waals (See Supplementary Fig. 2 ). Although the calculated results are consistent with the observed experiments, a relatively low Gibbs free energy for addition of NHC catalyst to the substrate suggests a rapid rate for this transformation. While the subsequent oxidative esterification is not the enantioselectivity-determined step, together with experimental obversion that increases the reaction temperature led to a higher enantioselectivity. 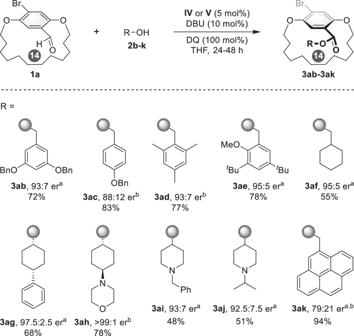Fig. 3: Evaluation of the effect of various alcohol substrates. aThe reaction was performed at room temperature,IVwas used as catalyst.bThe reaction was performed at 40 °C,Vwas used as catalyst. Thus, the Curtin-Hammet scenario might be operative for the DKR approach [55] . Fig. 9: Calculated energy profile. Calculated energy profile of the addition of NHC catalyst IV to [14]paracyclophane 1a . Full size image In summary, we developed an NHC-catalyzed enantioselective synthesis of planar-chiral cyclophanes. The reaction features a DKR process involving an aldehyde oxidation esterification and affords a wide range of planar-chiral macrocycles in good to high yields with high enantioselectivities. An investigation of ansa chain length and the size of aromatic ring substituents indicated that these variables were crucial to generating the planar chirality. Further, the cyclophane products could be transformed into other planar-chiral macrocyclic scaffolds by simple reactions. Controlled experiments and DFT calculations were performed to clarify the DKR process. An application of these planar-chiral scaffolds for library inclusion and asymmetric catalysis are under investigation in our lab. Materials. For 1 H NMR, 13 C NMR, and high-performance liquid chromatography spectra of compounds in this manuscript, see Supplementary Figures. For details of the synthetic macrocycle substrates: diphenol (10.0 mmol) and dibromides (10.0 mmol) in DMF (25.0 mL) were slowly added to a suspension of K 2 CO 3 (3.45 g, 25.0 mmol) and NaI (170 mg, 1.0 mmol) in DMF (150 mL) at 140 °C over 18 h. The solvent was removed under reduced pressure. The aqueous phase was extracted with EtOAc (3 × 50 mL), and the combined organic layers were washed with water and brine, and dried over Na 2 SO 4 . The solvent was removed under reduced pressure, and the residue was purified by flash column chromatography on silica gel affording the products (yield: 10 ~ 40%). Synthesis of 3 and 5 . To a 15 mL Schlenk tube equipped with a magnetic stirring bar was added macrocycles substrates 1 or 4 (0.10 mmol), 2 (0.4 mmol), NHC precursor IV or V (0.005 mmol), DBU (0.01 mmol) and DQ (0.1 mmol). 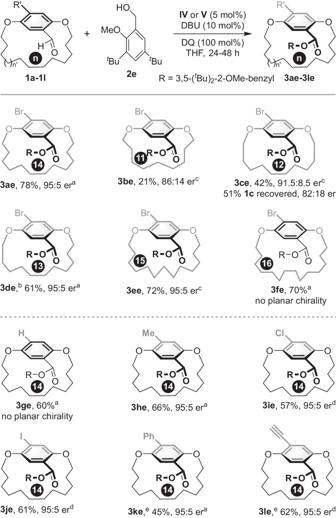Fig. 4: Evaluation of the ansa chain length and aromatic ring substituent size. aThe reaction was performed at room temperature,IVwas used as catalyst.bThe reaction was performed at 40 °C,Vwas used as catalyst.c0.2 mmol of2awas used.dThe reaction was performed at 50 °C,Vwas used as catalyst.eThe reaction was stirred at room temperature for 24 h,1kwas recovered in 55:45 er, and1 lwas recovered in 50:50 er. The tube was closed with a septum, evacuated, and refilled with nitrogen (3 cycles). Then, freshly distilled THF (1.0 mL) was added to the reaction mixture and stirred for 10–72 h. Upon completion (monitored by TLC), the solvent was evaporated, and the residue was purified by silica gel column chromatography to afford the planar-chiral cyclophanes 3 or 5 . 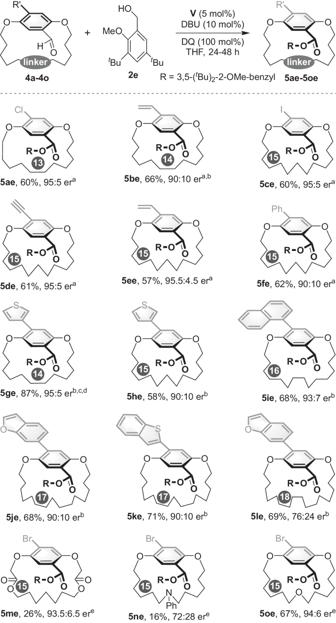Fig. 5: The scope of [n]paracyclophanes. aThe reaction was performed at 40 °C.bThe reaction was performed at 50 °C.cThe reaction was performed at room temperature,5gewas obtained in 86:14 er.dThe reaction was performed at 40 °C,5gewas obtained in 92:8 er.eThe reaction was performed at 40 °C,IVwas used as catalyst. 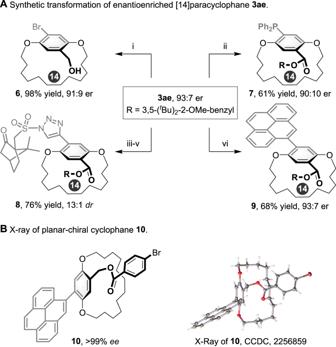Fig. 6: Derivatizations of the chiral product. ASynthetic transformation of enantioenriched [14]paracyclophane3ae. Reaction conditions: (i) LiAlH4, 0 °C, THF, 2 h. (ii) Ni(dppe)Cl2, Ph2PH, Et3N, DMF, 120 °C, 12 h. (iii) Pd(PPh3)2Cl2, CuI, TMS-acetylene, Et3N, 50 °C, 10 h, THF, 91% yield, 93:7 er. (iv) TBAF•3H2O, THF, rt, 4 h, 87% yield, 93:7 er. (v) CuTC, (R)-Camphor-10-sulfonyl azide, toluene, rt, 4 h, 96% yield, 13:1 dr. (vi) Pd(PPh3)4, Na2CO3, pyren-1-ylboronic acid, 1,4-dioxane, 100 °C, 24 h, 68% yield, 93:7 er.BX-ray of planar-chiral cyclophane10. 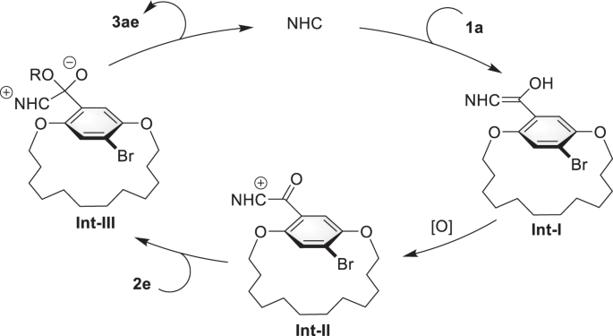Fig. 7 Postulated mechanism of the reaction. 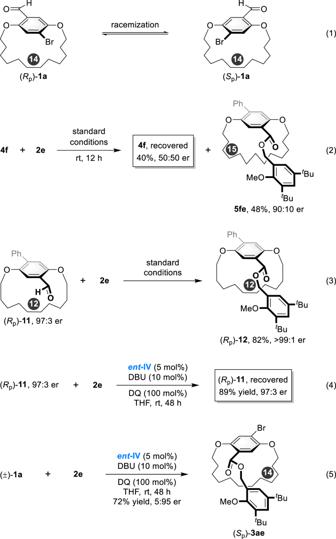Fig. 8 Controlled experiments of the dynamic kinetic resolution process. 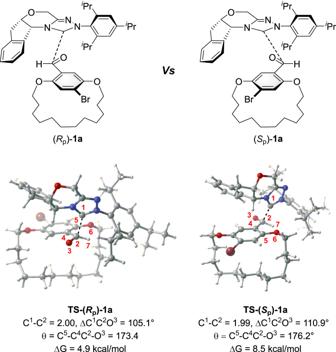Fig. 9: Calculated energy profile. Calculated energy profile of the addition of NHC catalystIVto [14]paracyclophane1a. Reporting summary Further information on research design is available in the Nature Portfolio Reporting Summary linked to this article.